Multiplex CRISPR/Cas9-based genome editing for correction of dystrophin mutations that cause Duchenne muscular dystrophy The CRISPR/Cas9 genome-editing platform is a promising technology to correct the genetic basis of hereditary diseases. The versatility, efficiency and multiplexing capabilities of the CRISPR/Cas9 system enable a variety of otherwise challenging gene correction strategies. Here, we use the CRISPR/Cas9 system to restore the expression of the dystrophin gene in cells carrying dystrophin mutations that cause Duchenne muscular dystrophy (DMD). We design single or multiplexed sgRNAs to restore the dystrophin reading frame by targeting the mutational hotspot at exons 45–55 and introducing shifts within exons or deleting one or more exons. Following gene editing in DMD patient myoblasts, dystrophin expression is restored in vitro. Human dystrophin is also detected in vivo after transplantation of genetically corrected patient cells into immunodeficient mice. Importantly, the unique multiplex gene-editing capabilities of the CRISPR/Cas9 system facilitate the generation of a single large deletion that can correct up to 62% of DMD mutations. Genome-editing technologies use synthetic nucleases to induce cellular DNA repair mechanisms and introduce site-specific, predefined genetic modifications in complex genomes [1] . These engineered enzymes are commonly based on zinc finger nucleases (ZFNs) [1] , transcription activator-like effector nucleases (TALENs) [2] , meganucleases [3] and most recently the RNA-guided CRISPR/Cas9 system [4] , [5] , [6] , [7] , [8] , [9] , [10] . The nucleases create site-specific double-strand breaks at predefined genomic sites that stimulate either non-homologous end joining (NHEJ) for targeted gene disruption or homologous recombination for highly efficient gene targeting. The simplicity and versatility of the CRISPR/Cas9 genome-editing system has led to rapid adoption and expansion of this technology that has proven to be remarkably robust for manipulating gene sequences in human cells. This has enabled new possibilities such as efficient multiplex gene editing for simultaneously inactivating multiple genes [5] , [6] , [11] . In this study, we apply the CRISPR system to repair genes mutated in hereditary disease, including capitalizing on the unique multiplex capacity of this technology to create large genomic deletions that restore gene expression. CRISPR/Cas9 systems have been adapted from multiple bacterial species, including Streptococcus pyogenes , S. thermophilus and Neisseria meningitidis , to efficiently generate targeted gene modifications in human cells [5] , [6] , [7] , [8] , [9] , [10] , [12] . These systems consist of a Cas9 nuclease that is co-expressed with a single guide RNA (sgRNA) molecule. Cas9 forms a complex with the 3′ end of the sgRNA, and the protein–RNA pair recognizes its genomic target by complementary base pairing between the 5′ end of the sgRNA sequence and a predefined 20 bp DNA sequence, known as the protospacer. By simply exchanging the 20-bp recognition sequence of the expressed sgRNA, the Cas9 nuclease can be directed to new genomic targets. The only restriction for protospacer targeting is that the sequence must be immediately followed by the protospacer-adjacent motif (PAM), a short sequence recognized by the Cas9 nuclease that is required for DNA cleavage. Several studies of the S. pyogenes CRISPR system have defined the PAM sequence for this Cas9 (SpCas9) as 5′-NGG-3′ and characterized the specificity of this system in human cells [13] , [14] , [15] , [16] , [17] , [18] , [19] . A unique capability of the CRISPR/Cas9 system is the straightforward ability to simultaneously target multiple distinct genomic loci by co-expressing a single Cas9 protein with two or more sgRNAs [5] , [6] , [11] , [20] . One of the most promising applications of genome editing is the correction of genetic mutations associated with hereditary disease [1] , [2] , [3] , [4] . Duchenne muscular dystrophy (DMD) is the most common hereditary disease; no effective treatments exist for this disorder. DMD is a severe X-linked disease that presents with progressive muscle wasting that typically leads to loss of ambulation in the second decade and death within the third decade of life because of respiratory complications or heart failure. The molecular basis of DMD is a mutation in the dystrophin gene [21] that leads to the complete lack of function of this essential skeletal muscle protein. These mutations are most commonly frameshifts generated by large intragenic deletions of one or more exons. DMD is the prototypical example of a group of monogenetic hereditary diseases that can be corrected by removing internal, but unessential, regions of the mutated gene to restore the proper reading frame [22] , [23] . For example, there is a class of common deletions in the exon 45–55 mutation hotspot region of the dystrophin gene that maintain the correct reading frame and lead to the expression of a truncated, but functional, dystrophin protein. Patients with this class of mutations are often asymptomatic or display mild symptoms associated with Becker muscular dystrophy, a substantially less severe disease than DMD. This has led to significant interest in developing an oligonucleotide-mediated exon skipping strategy that will restore the dystrophin reading frame during mRNA processing and convert DMD to a Becker-like phenotype [22] . Whereas early clinical trials in this area have focused on skipping exon 51 (refs 24 , 25 ), which is applicable to 13% of DMD patients, other preclinical efforts have demonstrated multi-exon skipping of the complete exon 45–55 coding region with a combination treatment of up to ten oligonucleotides [26] , [27] that could potentially address greater than 60% of known DMD patient mutations [23] . However, there are significant technical and practical hurdles to designing and developing this type of complex combination therapy, in addition to the general challenges of developing any oligonucleotide-based therapy that must be continuously administered for the lifetime of the patient. In contrast to these transient mRNA-targeted oligonucleotide-mediated exon skipping strategies, genome editing has the ability to make precise and permanent changes to gene sequences that will persist after cell division. In addition, only two nucleases are necessary to delete a genomic region of any length, in contrast to exon skipping in which a distinct oligonucleotide must be designed for each exon to be removed from the mRNA transcript. Genome editing using various designer nucleases has been proposed as a promising method to restore the native dystrophin gene in DMD patient cells [28] , [29] , [30] . However, an obstacle to implementing this approach has been successfully engineering the multiple nucleases targeted to the exons and introns necessary to address a large fraction of the DMD patient population. In this study, we take advantage of the versatility of the S. pyogenes CRISPR/Cas9 system to show proof-of-concept that this approach can rapidly and efficiently generate targeted frameshifts and large deletions to address commonly occurring mutations in the dystrophin gene across exons 45–55. Skeletal myoblasts from DMD patients were treated with sgRNAs and SpCas9 to correct patient-specific mutations and edited cells were enriched by fluorescence-activated cell sorting. Gene editing by CRISPR/Cas9 resulted in restored dystrophin mRNA transcripts and protein expression. Significantly, we generated a large deletion of 336 kb across a mutational hotspot containing exons 45–55 that is applicable to correction of greater than 60% of DMD patient mutations. This genomic deletion resulted in the loss of exons 45–55 in the corresponding dystrophin transcript and restored dystrophin expression in human DMD cells. In addition, an enriched pool of gene-corrected cells demonstrated expression of human dystrophin in vivo following engraftment into immunodeficient mice. CRISPR/Cas9 gene editing did not have significant toxic effects in human myoblasts as observed by stable gene editing frequencies and minimal cytotoxicity of several sgRNAs. However, gene-editing activity was confirmed at 3 out of 50 predicted off-target sites across five sgRNAs and CRISPR/Cas9-induced chromosomal translocations between on-target and off-target sites were detectable in immortalized cell lines. These data indicate a need to increase the specificity of this technology, although only a fraction of these events were detectable in the treated myoblasts from DMD patients. Collectively, this study provides proof-of-principle that the CRISPR/Cas9 technology is a versatile method for correcting a significant fraction of dystrophin mutations and with continued development may serve as a general platform for treating genetic disease. Targeting hotspot mutations in the human dystrophin gene To utilize the CRISPR/Cas9 gene-editing platform for correcting a wide range of dystrophin mutations, we created dozens of sgRNAs targeted to the hotspot mutation region between exons 45 and 55 ( Fig. 1 ). We selected the previously described S. pyogenes system that utilizes a human codon-optimized SpCas9 nuclease [5] , [6] and a chimeric single guide RNA (sgRNA) expression vector to direct efficient site-specific gene editing. Similar to our previous study targeting exon 51 with TALENs [28] , we selected protospacers to target the 5′ and 3′ ends of exons 45–55, which meet the 5′-NGG-3′ PAM requirement of SpCas9. Small insertions or deletions created by NHEJ-based DNA repair within these exons can generate targeted frameshift mutations that address various dystrophin mutations surrounding each exon ( Fig. 1a,b ). For example, CR3 was designed to correct dystrophin mutations or deletions surrounding exon 51 by introducing small insertions or deletions in the 5′ end of exon 51 to restore the downstream dystrophin reading frame ( Fig. 1b ). In addition, we designed sgRNAs to employ the multiplex capability of the CRISPR/Cas9 system and specifically delete individual exons or a series of exons to restore the dystrophin reading frame, similar to the methods of oligonucleotide-based exon skipping. For this purpose, sgRNAs were targeted to the intronic regions surrounding exon 51 ( Fig. 1c ) or exons 45–55 ( Fig. 1d ). These sgRNAs were intentionally targeted to sites nearest to the downstream or upstream exon intended to be included in the resulting transcript to minimize the likelihood that the background patient deletion would include the intronic sgRNA target sites. 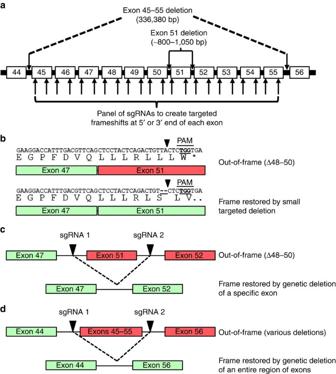Figure 1: CRISPR/Cas9 targeting of the dystrophin gene. (a) sgRNA sequences were designed to bind sequences in the exon 45–55 mutational hotspot region of the dystrophin gene, such that gene editing could restore dystrophin expression from a wide variety of patient-specific mutations. Arrows within introns indicate sgRNA targets designed to delete entire exons from the genome. Arrows within exons indicate sgRNA targets designed to create targeted frameshifts in the dystrophin gene. (b) Example of frame correction following introduction of small insertions or deletions by NHEJ DNA repair in exon 51 using the CR3 sgRNA. (c) Schematic of multiplex sgRNA targets designed to delete exon 51 and restore the dystrophin reading frame in a patient mutation with the deletion of exons 48–50. (d) Schematic of multiplex sgRNA targets designed to delete the entire exon 45–55 region to address a variety of DMD patient mutations. Figure 1: CRISPR/Cas9 targeting of the dystrophin gene. ( a ) sgRNA sequences were designed to bind sequences in the exon 45–55 mutational hotspot region of the dystrophin gene, such that gene editing could restore dystrophin expression from a wide variety of patient-specific mutations. Arrows within introns indicate sgRNA targets designed to delete entire exons from the genome. Arrows within exons indicate sgRNA targets designed to create targeted frameshifts in the dystrophin gene. ( b ) Example of frame correction following introduction of small insertions or deletions by NHEJ DNA repair in exon 51 using the CR3 sgRNA. ( c ) Schematic of multiplex sgRNA targets designed to delete exon 51 and restore the dystrophin reading frame in a patient mutation with the deletion of exons 48–50. ( d ) Schematic of multiplex sgRNA targets designed to delete the entire exon 45–55 region to address a variety of DMD patient mutations. Full size image Screening sgRNAs targeted to the human dystrophin gene We initially assessed gene-editing frequency in the human HEK293T cell line to rapidly determine different sgRNA targeting efficiencies. As quantified by the Surveyor assay 3 days post transfection, we found that 29 out of 32 (~90%) of sgRNAs tested were able to mediate efficient gene modification at the intended locus ( Table 1 and Supplementary Fig. 1 ). The gene-editing frequencies were stable for almost all of the sgRNAs (<25% signal change from day 3 to day 10, Table 1 and Supplementary Fig. 2 ), indicating that gene editing mediated by each individual sgRNA was well tolerated. An exception is CR33, which had no detectable activity at day 10, although activity may be below the sensitivity of the Surveyor assay (estimated ~1%). Table 1 Measured activity of sgRNAs in human cells. Full size table Enrichment of corrected cells We next sought to use selected sgRNAs to correct specific mutations in DMD patient myoblast cell lines. After transfection into DMD myoblasts, we observed unexpectedly low or undetectable gene modification activity as measured by the Surveyor assay ( Fig. 2c , bulk population). Therefore, we used flow cytometry to select for transfected cells co-expressing green fluorescent protein (GFP) through a 2A ribosomal skipping peptide linked to the SpCas9 protein ( Fig. 2a ), similar to previously described methods to enrich gene-modified cell populations using fluorescent reporters [31] , [32] . Importantly, the addition of this fluorescent reporter to the SpCas9 expression vector did not significantly impact gene-editing activity in HEK293T cells ( Fig. 2b ). A low percentage of transfected myoblasts (~0.5–2%) expressed the fluorescent reporter at 3 days after electroporation, despite high transfection efficiencies of a control GFP expression plasmid (typically >70%, Fig. 2d , pmaxGFP). Given the high levels of CRISPR/Cas9 activity in the easily transfected HEK293T cell line and previous studies demonstrating robust expression from the cytomegalovirus promoter in skeletal myoblasts, inefficient plasmid delivery by electroporation or vector-specific effects were likely responsible for the low observed gene editing efficiencies in unsorted cells. After sorting the GFP-positive DMD myoblasts, we observed a substantial increase in detectable activity at most sgRNA target loci ( Fig. 2c ). Therefore, all subsequent experiments used cells sorted for SpCas9 expression by expression of this fluorescent reporter. 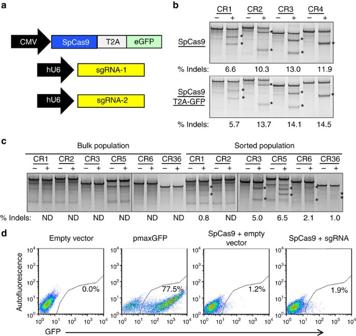Figure 2: Fluorescence-activated flow sorting to enrich genetically modified DMD myoblasts. (a) A plasmid expressing a human codon-optimized SpCas9 protein linked to a GFP marker using a T2A ribosomal skipping peptide sequence was co-electroporated into human DMD myoblasts with one or two plasmids carrying sgRNA expression cassettes. (b) The indicated sgRNA expression cassettes were independently co-transfected into HEK293T cells with a separate plasmid expressing SpCas9 with (bottom) or without (top) a GFP marker linked to SpCas9 by a T2A ribosomal skipping peptide sequence. Gene modification frequencies were assessed at 3 days post transfection by the Surveyor assay. Asterisks indicate cleaved PCR amplicon fragments at the expected sizes indicative of indels generated by gene editing. (c) DMD myoblasts with deletions of exons 48–50 in the dystrophin gene were treated with sgRNAs that correct the dystrophin reading frame in these patient cells. Gene modification was assessed at 20 days post-electroporation in unsorted (bulk) or GFP+sorted cells. (d) GFP expression in DMD myoblasts 3 days after electroporation with indicated expression plasmids. Transfection efficiencies and sorted cell populations are indicated by the gated region. ND, not determined. Figure 2: Fluorescence-activated flow sorting to enrich genetically modified DMD myoblasts. ( a ) A plasmid expressing a human codon-optimized SpCas9 protein linked to a GFP marker using a T2A ribosomal skipping peptide sequence was co-electroporated into human DMD myoblasts with one or two plasmids carrying sgRNA expression cassettes. ( b ) The indicated sgRNA expression cassettes were independently co-transfected into HEK293T cells with a separate plasmid expressing SpCas9 with (bottom) or without (top) a GFP marker linked to SpCas9 by a T2A ribosomal skipping peptide sequence. Gene modification frequencies were assessed at 3 days post transfection by the Surveyor assay. Asterisks indicate cleaved PCR amplicon fragments at the expected sizes indicative of indels generated by gene editing. ( c ) DMD myoblasts with deletions of exons 48–50 in the dystrophin gene were treated with sgRNAs that correct the dystrophin reading frame in these patient cells. Gene modification was assessed at 20 days post-electroporation in unsorted (bulk) or GFP + sorted cells. ( d ) GFP expression in DMD myoblasts 3 days after electroporation with indicated expression plasmids. Transfection efficiencies and sorted cell populations are indicated by the gated region. ND, not determined. Full size image Restoration of dystrophin expression by targeted frameshifts We have shown previously that small insertions and deletions created by NHEJ DNA repair can be used to create targeted frameshifts to correct aberrant reading frames [28] . Similar to this approach, we designed a sgRNA, CR3, to restore the dystrophin reading frame by introducing small insertions and deletions within exon 51 ( Figs 1b and 3a ). The types of insertions and deletions generated by CRISPR/Cas9 at this locus were assessed by Sanger sequencing of alleles from the genomic DNA of HEK293T cells co-transfected with expression plasmids for SpCas9 and the CR3 sgRNA ( Fig. 3b ). Notably, the insertions and deletions resulted in conversion to all three reading frames ( Fig. 3b,c ), consistent with our previous results using TALENs [28] . To demonstrate genetic correction in a relevant patient cell line, expression plasmids for SpCas9 and the CR3 sgRNA were electroporated into DMD myoblasts with a deletion of exons 48–50 that is correctable by creating frameshifts in exon 51. The treated cells were sorted, verified to have gene modification activity by the Surveyor assay (CR3, Fig. 2c sorted population), and differentiated into myotubes to test for restored dystrophin expression. Expression of dystrophin protein was observed concomitant with the detectable nuclease activity ( Fig. 3d and Supplementary Fig. 4 ). Taken together with the data from Table 1 , the S. pyogenes CRISPR/Cas9 system presents a powerful method to quickly generate targeted frameshifts to address a variety of patient mutations and restore expression of the human dystrophin gene. 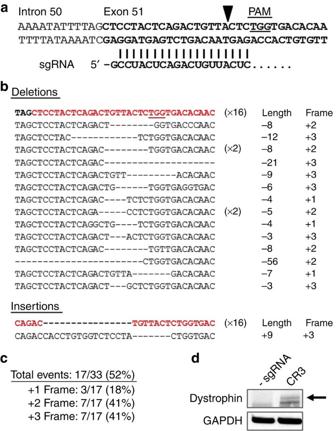Figure 3: Targeted frameshifts to restore the dystrophin reading frame using CRISPR/Cas9. (a) The 5′ region of exon 51 was targeted using a sgRNA, CR3, that binds immediately upstream of the first out-of-frame stop codon. PAM: protospacer-adjacent motif. (b) The exon 51 locus was PCR amplified from HEK293T cells treated with SpCas9 and CR3 expression cassettes. Sequences of individual clones were determined by Sanger sequencing. The top sequence (bolded, exon in red) is the native, unmodified sequence. The number of clones for each sequence is indicated in parentheses. (c) Summary of total gene editing efficiency and reading frame conversions resulting from gene modification shown inb. (d) Western blot for dystrophin expression in human DMD myoblasts treated with SpCas9 and the CR3 sgRNA expression cassette (Fig. 2c) to create targeted frameshifts to restore the dystrophin reading frame. Dystrophin expression was probed using an antibody against the rod-domain of the dystrophin protein after 6 days of differentiation. Figure 3: Targeted frameshifts to restore the dystrophin reading frame using CRISPR/Cas9. ( a ) The 5′ region of exon 51 was targeted using a sgRNA, CR3, that binds immediately upstream of the first out-of-frame stop codon. PAM: protospacer-adjacent motif. ( b ) The exon 51 locus was PCR amplified from HEK293T cells treated with SpCas9 and CR3 expression cassettes. Sequences of individual clones were determined by Sanger sequencing. The top sequence (bolded, exon in red) is the native, unmodified sequence. The number of clones for each sequence is indicated in parentheses. ( c ) Summary of total gene editing efficiency and reading frame conversions resulting from gene modification shown in b . ( d ) Western blot for dystrophin expression in human DMD myoblasts treated with SpCas9 and the CR3 sgRNA expression cassette ( Fig. 2c ) to create targeted frameshifts to restore the dystrophin reading frame. Dystrophin expression was probed using an antibody against the rod-domain of the dystrophin protein after 6 days of differentiation. Full size image Multiplex CRISPR/Cas9 gene editing to delete exon 51 The multiplexing capability of the CRISPR/Cas9 system presents a novel method to efficiently generate genomic deletions of specific exons for targeted gene correction. DMD patient myoblasts with background deletions correctable by exon 51 skipping were treated with two combinations of sgRNAs flanking exon 51 (CR1/CR5 or CR2/CR5) and sorted to enrich for gene-edited cells as in Fig. 2 . As detected by end-point PCR of the genomic DNA from these treated cells, the expected genomic deletions were only present when both sgRNAs were electroporated into the cells with SpCas9 ( Fig. 4a ). Sanger sequencing confirmed the expected junction of the distal chromosomal segments ( Fig. 4b ) for both deletions. After differentiating the sorted myoblasts, a deletion of exon 51 from the mRNA transcript was detected only in the cells treated with both sgRNAs ( Fig. 4c ). Finally, restored dystrophin protein expression was detected in the treated cells concomitant with observed genome- and mRNA-level deletions of exon 51 ( Fig. 4d and Supplementary Fig. 4 ). 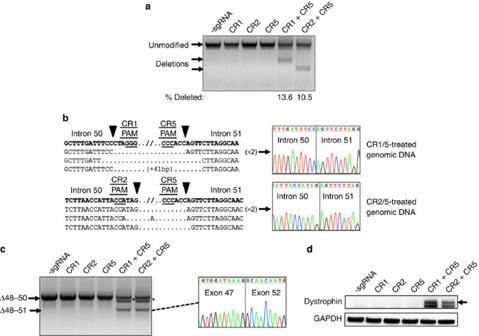Figure 4: Deletion of exon 51 from the human genome using multiplex CRISPR/Cas9 gene editing. (a) End-point genomic PCR across the exon 51 locus in human DMD myoblasts with a deletion of exons 48–50. The top arrow indicates the expected position of full-length PCR amplicons and the two lower arrows indicate the expected position of PCR amplicons with deletions caused by the indicated sgRNA combinations. (b) PCR products fromawere cloned and individual clones were sequenced to determine insertions and deletions present at the targeted locus. The top row shows the wild-type unmodified sequence and the triangles indicate SpCas9 cleavage sites. At the right are representative chromatograms showing the sequences of the expected deletion junctions. (c) End-point reverse transcription–PCR analysis of dystrophin mRNA transcripts in CRISPR/Cas9-modified human Δ48–50 DMD myoblasts treated with the indicated sgRNAs. A representative chromatogram of the expected deletion PCR product is shown at the right. Asterisk: band resulting from hybridization of the deletion product strand to the unmodified strand. (d) Rescue of dystrophin protein expression by CRISPR/Cas9 genome editing was assessed by western blot for the dystrophin protein with GAPDH as a loading control. The arrow indicates the expected restored dystrophin protein band. Figure 4: Deletion of exon 51 from the human genome using multiplex CRISPR/Cas9 gene editing. ( a ) End-point genomic PCR across the exon 51 locus in human DMD myoblasts with a deletion of exons 48–50. The top arrow indicates the expected position of full-length PCR amplicons and the two lower arrows indicate the expected position of PCR amplicons with deletions caused by the indicated sgRNA combinations. ( b ) PCR products from a were cloned and individual clones were sequenced to determine insertions and deletions present at the targeted locus. The top row shows the wild-type unmodified sequence and the triangles indicate SpCas9 cleavage sites. At the right are representative chromatograms showing the sequences of the expected deletion junctions. ( c ) End-point reverse transcription–PCR analysis of dystrophin mRNA transcripts in CRISPR/Cas9-modified human Δ48–50 DMD myoblasts treated with the indicated sgRNAs. A representative chromatogram of the expected deletion PCR product is shown at the right. Asterisk: band resulting from hybridization of the deletion product strand to the unmodified strand. ( d ) Rescue of dystrophin protein expression by CRISPR/Cas9 genome editing was assessed by western blot for the dystrophin protein with GAPDH as a loading control. The arrow indicates the expected restored dystrophin protein band. Full size image Dystrophin rescue by a multi-exon large genomic deletion Although addressing patient-specific mutations is a powerful use of the CRISPR/Cas9 system, it would be advantageous to develop a single method that can address a myriad of common patient deletions. For example, a promising strategy is to exclude the entire exon 45–55 region as a method to correct up to 62% of known patient deletions [22] , [26] , [27] . Therefore, we tested if multiplex CRISPR/Cas9-based gene editing may be able to generate efficient deletion of the exon 45–55 locus in human cells. After transfection into HEK293T cells, we detected the expected deletion of ~336,000 bp by PCR of the genomic DNA ( Fig. 5a ). Similarly, we were able to detect this deletion by PCR of the genomic DNA from SpCas9/sgRNA-treated DMD patient cells harbouring a background deletion of exons 48–50 of unknown length ( Fig. 5a ). Sanger sequencing of this deletion band from the genomic DNA of treated DMD cells revealed the expected junctions of intron 44 and intron 55 immediately adjacent to the sgRNA target sites ( Fig. 5b ). After differentiation of treated DMD cells, the expected deletion of exons 45–55 was detected in the dystrophin mRNA transcript and verified to be a fusion of exons 44 and 56 by Sanger sequencing ( Fig. 5c ). Based on the intensity of the modified mRNA band compared with the unmodified band, the efficiency of this 336 kb deletion was less than the efficiency of exon 51 deletion ( Fig. 4a,c ), which is expected based on previous studies showing a size-dependent decrease in the efficiency of nuclease-mediated genomic deletions [20] , [33] . Nevertheless, restored protein expression was observed by western blot in the sorted cell populations containing the CRISPR/Cas9-induced deletion of exons 45–55 from the genome and resulting mRNA transcripts ( Fig. 5d and Supplementary Fig. 4 ). These data demonstrate that multiplex CRISPR/Cas9 editing presents a single universal method to restore the dystrophin reading frame in more than 60% of DMD patient mutations. 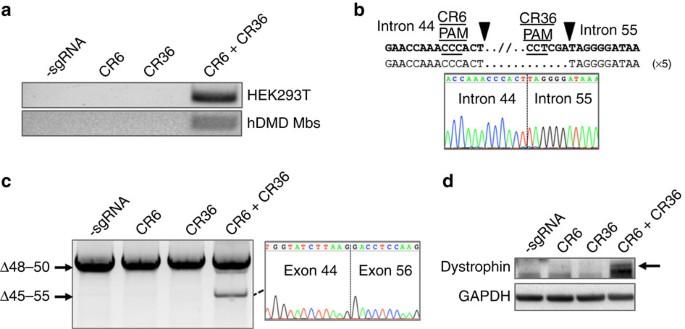Figure 5: Deletion of the exon 45–55 region in human DMD myoblasts by multiplex CRISPR/Cas9 gene editing. (a) End-point PCR of genomic DNA to detect deletion of the region between intron 44 and intron 55 after treating HEK293T cells or DMD myoblasts with the indicated sgRNAs. (b) Individual clones of PCR products of the expected size for the deletions from DMD myoblasts inawere analysed by Sanger sequencing to determine the sequences of genomic deletions present at the targeted locus. Below is a representative chromatogram showing the sequence of the expected deletion junctions. (c) End-point reverse transcription–PCR analysis of dystrophin mRNA transcripts in CRISPR/Cas9-modified human Δ48–50 DMD myoblasts treated with the indicated sgRNAs. A representative chromatogram of the expected deletion PCR product is shown at the right. (d) Analysis of restored dystrophin protein expression by western blot following electroporation of DMD myoblasts with sgRNAs targeted to intron 44 and/or intron 55. Figure 5: Deletion of the exon 45–55 region in human DMD myoblasts by multiplex CRISPR/Cas9 gene editing. ( a ) End-point PCR of genomic DNA to detect deletion of the region between intron 44 and intron 55 after treating HEK293T cells or DMD myoblasts with the indicated sgRNAs. ( b ) Individual clones of PCR products of the expected size for the deletions from DMD myoblasts in a were analysed by Sanger sequencing to determine the sequences of genomic deletions present at the targeted locus. Below is a representative chromatogram showing the sequence of the expected deletion junctions. ( c ) End-point reverse transcription–PCR analysis of dystrophin mRNA transcripts in CRISPR/Cas9-modified human Δ48–50 DMD myoblasts treated with the indicated sgRNAs. A representative chromatogram of the expected deletion PCR product is shown at the right. ( d ) Analysis of restored dystrophin protein expression by western blot following electroporation of DMD myoblasts with sgRNAs targeted to intron 44 and/or intron 55. Full size image Transplantation of corrected myoblasts into mice A potential strategy for DMD therapy is to correct a population of autologous patient muscle progenitor cells that can be engrafted into the patient’s skeletal muscle tissue to rescue dystrophin expression [34] , [35] , [36] , [37] , [38] , [39] , [40] . To demonstrate the ability of the corrected cells to express correctly localized human dystrophin in vivo , we transplanted a population of DMD myoblasts that were treated with sgRNAs CR1 and CR5, which flank exon 51, and sorted for expression of GFP as before ( Figs 2 and 4 and Supplementary Fig. 3 ). After 4 weeks, muscle fibres positive for human spectrin, which is expressed by both corrected and uncorrected cells, were detected in cryosections of injected muscle tissue ( Fig. 6 ). Several of these fibres were also positive for human dystrophin with expression properly localized to the sarcolemma, indicating correct function of the restored protein ( Fig. 6 and Supplementary Fig. 5 ). The frequency of dystrophin-positive fibres was low, potentially due to the effects of electroporation, extensive culture and sorting, the efficiency of editing ( Fig. 4a and Supplementary Fig. 3 ), overall dystrophin expression levels and/or the quality of available antibodies. Nevertheless, fibres positive for both spectrin and dystrophin were found across several sections in multiple injected mice ( Fig. 6 and Supplementary Fig. 5 ), validating consistent in vivo expression of the restored protein in a fraction of implanted cells. Importantly, no fibres positive for human dystrophin were observed in any sections from mice injected with the untreated DMD myoblasts, confirming that the CRISPR/Cas9-modified cells were the source of human dystrophin expression. 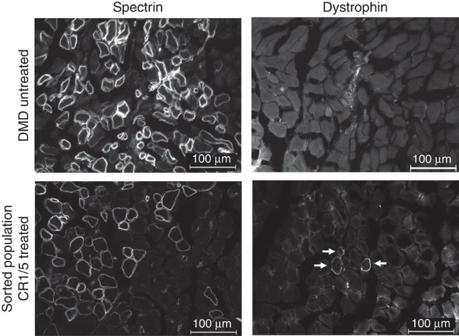Figure 6: Expression of restored human dystrophinin vivofollowing cell transplantation. Human Δ48–50 DMD myoblasts were treated with SpCas9, CR1 and CR5 to delete exon 51 and sorted for GFP expression as shown inFig. 2. These sorted cells and untreated control cells were injected into the hind limbs of immunodeficient mice and assessed for human-specific protein expression in muscle fibres after 4 weeks post transplantation. Cryosections were stained with anti-human spectrin, which is expressed by both uncorrected and corrected myoblasts that have fused into mouse myofibers, or anti-human dystrophin antibodies as indicated. White arrows indicate muscle fibres positive for human dystrophin. Scale bars indicate 100 μm. ND, not determined. Figure 6: Expression of restored human dystrophin in vivo following cell transplantation. Human Δ48–50 DMD myoblasts were treated with SpCas9, CR1 and CR5 to delete exon 51 and sorted for GFP expression as shown in Fig. 2 . These sorted cells and untreated control cells were injected into the hind limbs of immunodeficient mice and assessed for human-specific protein expression in muscle fibres after 4 weeks post transplantation. Cryosections were stained with anti-human spectrin, which is expressed by both uncorrected and corrected myoblasts that have fused into mouse myofibers, or anti-human dystrophin antibodies as indicated. White arrows indicate muscle fibres positive for human dystrophin. Scale bars indicate 100 μm. ND, not determined. Full size image Off-target and cytotoxicity analysis We assessed the relative cytotoxicity of the CRISPR/Cas9 system in human cells to a subset of sgRNAs by adapting a flow cytometry-based GFP retention assay as previously described [28] . Minimal cytotoxicity was observed for SpCas9 co-expressed with or without sgRNAs after transfection into human cells ( Fig. 7a ). Several recent studies have documented activity of the CRISPR/Cas9 system at off-target loci in human cells [13] , [14] , [15] , [16] , [17] , [18] , [19] . Public tools are available to assess and prioritize potential CRISPR/Cas9 activity at off-target loci based on predicted positional bias of a given mismatch in the sgRNA protospacer sequence and the total number of mismatches to the intended target site [14] . We used this public webserver to predict the most likely off-target sites for the sgRNAs used to correct the dystrophin gene in this study ( Supplementary Table 2 ). The top ten potential off-target sites (OT1 to OT10) were first assessed by the Surveyor assay in treated HEK293T cells because off-target activity in this cell line is well-known to be readily detectable due to high levels of transfection and expression of Cas9 and sgRNAs [13] , [14] , [15] , [16] , [17] , [18] , [19] and thus it would serve as a more rigorous test of specificity. We tested HE293T cells treated with SpCas9 and individual sgRNA expression cassettes for CR1, CR3, CR5, CR6 or CR36, for a total of 5 on-target and 50 off-target sites. For CR1, CR3 and CR36, one of the ten predicted off-target loci had significant levels of gene modification ( Supplementary Table 2 and Supplementary Fig. 6 ), consistent with other studies investigating the specificity of the S. pyogenes CRISPR/Cas9 system [13] , [14] , [15] , [16] , [17] , [18] . Interestingly, the CR3 off-target sequence had substantial homology and similar modification frequencies to the intended on-target (9.3% at OT1 versus 13.3% at intended site; Supplementary Table 2 and Supplementary Fig. 6 ). Notably, CR3-OT1 was the only one of these three off-target sites to show significant levels of activity in the sorted DMD myoblasts by the Surveyor assay ( Fig. 7b ). 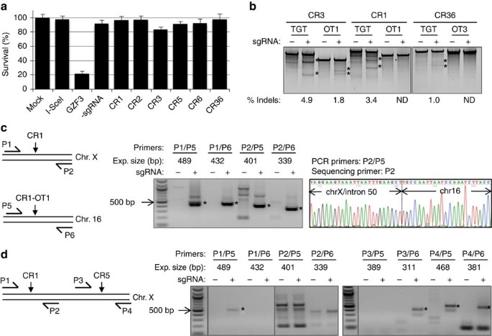Figure 7: Evaluation of CRISPR/Cas9 toxicity and off-target effects for deletion of human exon 51. (a) Results of a cytotoxicity assay in HEK293T cells treated with human-optimized SpCas9 and the indicated sgRNA constructs. Cytotoxicity is based on survival of GFP-positive cells that are co-transfected with the indicated nuclease. I-SceI is a well-characterized non-toxic meganuclease and GZF3 is a known toxic zinc finger nuclease.n=3 independent transfections (mean+s.e.m.). (b) Surveyor analysis at off-target sites in sorted hDMD cells treated with expression cassettes encoding SpCas9 and the indicated sgRNAs. These three off-target sites tested in hDMD cells were identified from a panel of 50 predicted sites tested in HEK293T cells (Supplementary Fig. 6andSupplementary Table 2). ND, not determined; OT, off-target locus; TGT, on-target locus for indicated sgRNA. (c,d) End-point nested PCR to detect chromosomal translocations in (c) HEK293T cells treated with Cas9 and CR1 or (d) sorted hDMD cells treated with Cas9, CR1 and CR5. The schematic depicts the relative location of nested primer pairs customized for each translocation event. The expected size of each band was estimated based on the primer size and the location of the predicted sgRNA cut site at each locus. Asterisks indicate bands detected at the expected size. The identities of the bands incwere verified by Sanger sequencing from each end (Supplementary Fig. 11). A representative chromatogram for the P2/P5 translocation in HEK293T cells is shown. Figure 7: Evaluation of CRISPR/Cas9 toxicity and off-target effects for deletion of human exon 51. ( a ) Results of a cytotoxicity assay in HEK293T cells treated with human-optimized SpCas9 and the indicated sgRNA constructs. Cytotoxicity is based on survival of GFP-positive cells that are co-transfected with the indicated nuclease. I-SceI is a well-characterized non-toxic meganuclease and GZF3 is a known toxic zinc finger nuclease. n =3 independent transfections (mean+s.e.m.). ( b ) Surveyor analysis at off-target sites in sorted hDMD cells treated with expression cassettes encoding SpCas9 and the indicated sgRNAs. These three off-target sites tested in hDMD cells were identified from a panel of 50 predicted sites tested in HEK293T cells ( Supplementary Fig. 6 and Supplementary Table 2 ). ND, not determined; OT, off-target locus; TGT, on-target locus for indicated sgRNA. ( c , d ) End-point nested PCR to detect chromosomal translocations in ( c ) HEK293T cells treated with Cas9 and CR1 or ( d ) sorted hDMD cells treated with Cas9, CR1 and CR5. The schematic depicts the relative location of nested primer pairs customized for each translocation event. The expected size of each band was estimated based on the primer size and the location of the predicted sgRNA cut site at each locus. Asterisks indicate bands detected at the expected size. The identities of the bands in c were verified by Sanger sequencing from each end ( Supplementary Fig. 11 ). A representative chromatogram for the P2/P5 translocation in HEK293T cells is shown. Full size image Deep sequencing of on-target and off-target sites was also used to quantify gene-editing activity with greater sensitivity. Similar to the strategy with the Surveyor assay, we first screened the 5 on-target and all 50 off-target sites in HEK293T cells ( Table 2 and Supplementary Table 3 ). Notably, the indel frequencies measured by deep sequencing were significantly greater than those determined by the Surveyor assay ( Table 1 ), suggesting the Surveyor assay may underestimate overall gene editing activity. The detection limit for activity by deep sequencing was ~0.01–0.1% indel-modified alleles, in contrast to ~1% by the Surveyor assay. Off-target sites were classified by greater than 0.2% indels or a tenfold increase in indels compared with control. By this independent method, the same three off-target sites were identified by deep sequencing as by the Surveyor assay. These three off-target sites and their corresponding on-target sites were also assayed in the sorted, treated DMD myoblasts and only one of the sites showed detectable levels of activity, at a frequency approximately one-third of on-target activity ( Table 2 and Supplementary Table 4 ). Thus, our selected sgRNAs have relatively favourable specificities, however, we cannot rule out activity at predicted off-target loci that may exist below the sensitivity of these assays or off-target activity at other loci that were not assessed here. Notably, these sequencing results also showed a strong preference for single base-pair insertions, consistent with previous studies [41] , as well as enrichment for specific indels that are likely mediated by microhomology at the DNA break [42] and could be used to favour conversion to specific reading frames ( Supplementary Figs 7 and 8 ). Table 2 On-target and off-target gene-editing activity by deep sequencing. Full size table Nuclease activity at off-target sites may cause unintended chromosomal rearrangements by distal re-ligation between cleaved target and off-target loci on distinct chromosomes [19] , [43] . This presents a significant concern for deletion-based gene correction strategies because of the increased potential for off-target activity by using two or more nucleases, such as in multiplex CRISPR/Cas9 gene editing. We probed for potential translocations using a highly sensitive nested genomic PCR assay to detect translocations at the validated off-target loci ( Table 2 and Supplementary Table 2 ) during both single and multiplex CRISPR/Cas9-editing strategies. Using this assay, we readily detected translocations between on-target and off-target sites in the model HEK293T cell line that also shows higher levels of off-target activity ( Fig. 7c and Supplementary Fig. 9a,b ). Sanger sequencing of the PCR amplicons confirmed the identity of the predicted translocation event for each primer pair ( Supplementary Figs 10 and 11 ). A subset of the translocations detected in the HEK293T cells were also detectable by nested PCR in the sorted hDMD myoblasts, although the signal was considerably weaker and we were unable to confirm the sequence identity due to low yield of product ( Fig. 7d and Supplementary Fig. 9a,c ). Notably, we did not detect translocations using this assay in HEK293T cells or sorted DMD myoblasts treated with CR36 or CR6/CR36, respectively ( Supplementary Fig. 9 ), that had low levels of off-target activity at CR36-OT3 only in HEK293T cells ( Table 2 and Supplementary Table 2 ). These results underscore the importance of selecting highly specific sgRNAs, particularly for multiplex editing applications, and show that this approach can benefit from ongoing efforts to improve the specificity of the CRISPR/Cas9 system [4] , [15] , [18] , [19] , [44] , [45] , [46] . However, taken together with the cytotoxicity and stable gene-editing activities observed in Table 1 , these data suggest that the selected sgRNAs are able to correct the dystrophin gene without significant toxicity and with only a single strongly predicted off-target site with detectable levels of activity. Genome editing is a powerful tool for correcting genetic disease and the recent development of the CRISPR/Cas9 system is dramatically accelerating progress in this area. A recent study showed the correction of the dystrophic phenotype in a mouse model of DMD by gene editing with CRISPR in single-cell mouse embryos [47] . Here we demonstrate the use of CRISPR to correct mutations to the human dystrophin gene in DMD patient cells. Many gene- and cell-based therapies for DMD are in preclinical development and clinical trials, and genome editing methods are compatible with many of these approaches. For example, genome editing may be combined with patient-specific cell-based therapies for DMD. Although transplantation of skeletal myoblasts, as used in this study, has been generally unsuccessful in clinical trials because of poor cell survival, engraftment, distribution and reconstitution of the progenitor cell population, several other muscle progenitor cells and pluripotent cell sources are currently under investigation and represent a potential path for this approach moving forward [34] , [35] , [36] , [37] , [38] , [39] , [40] . In fact, the CRISPR/Cas9 system has been previously demonstrated to function in human stem cells [9] , [10] , [48] and other human cell lines [5] , [6] , [7] , [8] , as well as human skeletal myoblasts in this study. Gene editing with CRISPR/Cas9 has also recently been achieved in vivo following plasmid delivery to the mouse liver [49] and AAV delivery to the brain [50] . Furthermore, genome editing of autologous primary T cells with ZFNs is currently in clinical trials (NCT01252641, NCT00842634 and NCT01044654) [51] . Importantly, gene editing with CRISPR/Cas9 did not abolish the myogenic capacity of the transfected myoblasts, as demonstrated by robust dystrophin expression in vitro and in vivo after transplantation into immunodeficient mice. Thus, this strategy should be compatible with cell-based therapies for DMD that are under development [34] , [35] , [36] , [37] , [38] , [39] , [40] , including induced pluripotent stem cells [37] , [38] , [39] that will likely provide a means to enhance the low engraftment efficiencies observed here with extensively cultured myoblasts ( Fig. 6 ). In addition, direct transfection of the sgRNA and Cas9 mRNA or protein to cultured cells, in contrast to the plasmid-based delivery method used here, may increase specificity and safety by reducing the duration of Cas9 expression and eliminating the possibility of random plasmid integration [52] , [53] . Delivery of Cas9 and the sgRNAs to cultured cells with non-integrating viral vectors, rather than electroporation, may also improve cell health, engraftment efficiency and in vivo dystrophin expression [54] , [55] . Alternatively, delivery of the CRISPR/Cas9 system directly to skeletal and/or cardiac muscle by viral, plasmid or RNA delivery vectors is a promising strategy for in vivo genome editing and translation of this approach [35] , [49] , [56] , [57] , [58] , [59] . The large size of S. pyogenes Cas9 gene (~4.2 kb) presents a challenge to its use in size-restricted adeno-associated viral vectors with typical constitutive or muscle-specific promoters. However, Cas9 genes from other species [12] , [60] , such as N. meningitidis and S. thermophilus , are small enough to efficiently package both Cas9 and sgRNA expression cassettes into single AAV vectors for in vivo gene-editing applications, as has been done with the smaller ZFNs [61] , [62] . The S. pyogenes CRISPR/Cas9 system enabled efficient modification of nearly 90% of tested targets, consistent with other reports of robust activity of this system at diverse loci. The robustness and versatility of this technology is a significant advancement towards at-will creation of patient-specific gene editing. However, further enhancing gene editing frequencies and minimizing off-target activity remain major challenges to customized clinical applications. Notably, recent studies have shown that low levels of dystrophin, including as little as 4% of wild-type expression, are sufficient to improve survival, motor function and cardiac function in a mouse model [63] , [64] , [65] . Therefore, the levels of gene editing reported in this study and others for primary human cells, often in the range of 5–10% edited alleles, may be sufficient for therapeutic benefit for this disease, particularly if using efficient in vivo delivery methods [57] , [58] or a robust progenitor cell source [34] , [35] , [36] , [37] , [38] , [39] , [40] for an ex vivo strategy. Regardless, we suspect that optimized delivery and expression vehicles, as well as ongoing improvements to the CRISPR/Cas9 system [4] , will lead to significant enhancements of gene correction levels. The use of multiplexing with CRISPR/Cas9 to delete exons also presents a unique set of opportunities and challenges. This is the first study to report the deletion of complete exons from the genome to restore dystrophin expression, in contrast to previous genome editing efforts that restored the reading frame of the dystrophin gene with small indels generated by NHEJ-based DNA repair following the action of a single nuclease [28] , [30] , inserted missing exons into the gene by homologous recombination [29] or inserted a microdystrophin expression cassette into a safe harbour site by homologous recombination [55] . A primary benefit of this new approach is that NHEJ is an active DNA repair mechanism in all cell types, whereas homologous recombination is typically only active in mitotic cells. As a result, approaches dependent on homologous recombination may not be applicable to directly modifying skeletal muscle fibres, although recent evidence of genome editing in the adult liver provides some support that this may be possible [49] , [61] . Another advantage of the current method, relative to the indel-based approach, is that the protein product of the edited gene is predictable and already characterized in Becker muscular dystrophy patients with the naturally occurring deletion. This is in contrast to the random indels created by intraexonic action of a single nuclease that will lead to the creation of novel epitopes from each DNA repair event. Furthermore, the product resulting from the exon deletions will lead to restored dystrophin for every successful gene editing event, whereas modifying the gene with random indels within exons will only restore the reading frame in the one-third of editing events that leads to the correct reading frame. Additional studies on enhancing and/or biasing gene repair towards distal chromosomal re-ligation will be helpful, particularly for long deletions such as the excision of the 336 kb containing exons 45–55 demonstrated in this study. Moreover, the introduction of multiple double-strand breaks increases the requirement for stringent specificity of the gene editing reagents in order to minimize the opportunity for the unintended chromosomal rearrangements that were readily detected in the treated HEK293T cells ( Fig. 7c,d and Supplementary Figs 9–11 ), but were less evident in the more relevant DMD myoblasts. We observed that all of the sgRNAs tested were not associated with significant cytotoxic effects in human cells. We identified three potential off-target sites out of 50 total tested sites for the five sgRNAs used here to restore dystrophin expression ( Table 2 and Supplementary Table 2 ). Furthermore, chromosomal translocations between the intended on-target sites and these off-target sites were detectable by highly sensitive nested PCR assays in HEK293T cells expressing high levels of Cas9 and sgRNAs. This is consistent with previous work showing translocations with two nucleases intentionally targeted to distinct chromosomes [43] . These results are also consistent with other studies that have characterized off-target activity and translocations generated by SpCas9 (refs 13 , 14 , 15 , 16 , 17 , 18 , 19 ) and compare favourably with other gene-editing systems, including ZFNs and TALENs, which are sometimes cytotoxic [66] and are known to also act at off-target sites [67] , [68] . Notably, the off-target activity and translocations identified in HEK293T cells, which is an immortalized and aneuploid cell line that expresses very high levels of Cas9 and sgRNA, did not occur at as high a level and in some cases were undetectable in the DMD myoblasts even though they were sorted for Cas9 expression ( Table 2 ). This corroborates previous studies showing that lower levels of Cas9 and sgRNA can reduce off-target effects [14] , [16] . Importantly, this level of specificity may be tolerable given the severity of DMD, the lack of an apparent cytotoxic effect in human cells, and the absence of adverse events in ongoing clinical trials for genome editing with ZFNs (NCT01252641, NCT00842634 and NCT01044654) [51] . Furthermore, improvements to the specificity of the CRISPR/Cas9 system, including the use of dual nickases, truncated sgRNAs, fusions to a FokI endonuclease domain, and careful sgRNA selection methods [15] , [18] , [19] , [44] , [45] , [46] , are also under development. CRISPR/Cas9 specificity may be further enhanced by rational design or directed evolution of the S. pyogenes sgRNA and/or Cas9 nuclease, or characterization of novel Cas9 nucleases from other species with more stringent sgRNA or PAM requirements [12] , [60] . This study demonstrates that CRISPR/Cas9 genome editing is a robust, easily programmable method to rapidly generate targeted frameshifts or genomic deletions that can address a variety of dystrophin mutations. Importantly, this method can reproducibly modify the dystrophin gene by deleting exons 45–55, thereby addressing more than half of DMD patient deletions with a single genome-editing strategy. Further advancements in the delivery, specificity and efficiency of these reagents will enhance the utility of this method for correcting the dystrophin gene and creating other custom genetic modifications. Thus, CRISPR/Cas9 genome editing offers an exciting new avenue for gene therapies to treat Duchenne muscular dystrophy and other hereditary disorders. Plasmid constructs The expression cassettes for the S. pyogenes sgRNA and human codon-optimized Cas9 (hCas9) nuclease were used as previously described [69] . In order to create a fluorescent reporter system to enrich CRISPR/Cas9-modified cells, a GeneBlock (IDT) was synthesized containing a portion of the 3′ end of the Cas9-coding sequence fused to a T2A skipping peptide immediately upstream of a multiple cloning site and subsequently cloned into the hCas9 expression vector. An eGFP reporter gene was then cloned into the T2A vector to allow co-translation of Cas9 and eGFP proteins from the same expression vector (hCas9-T2A-GFP, Supplementary Fig. 12 ). Cell culture and transfection HEK293T cells were obtained from the American Tissue Collection Center through the Duke Cell Culture Facility and were maintained in DMEM supplemented with 10% fetal bovine calf serum and 1% penicillin/streptomycin. Immortalized myoblasts [70] from a DMD patient harbouring a deletion of exons 48–50 (Δ48–50) in the dystrophin gene were maintained in skeletal muscle media (PromoCell) supplemented with 20% fetal bovine calf serum (Sigma), 50 μg ml −1 fetuin, 10 ng ml −1 human epidermal growth factor (Sigma), 1 ng ml −1 human basic fibroblast growth factor (Sigma), 10 μg ml −1 human insulin (Sigma), 1% GlutaMAX (Invitrogen) and 1% penicillin/streptomycin (Invitrogen). All cell lines were maintained at 37 °C and 5% CO 2 . HEK293T cells were transfected with Lipofectamine 2000 (Invitrogen) with 400 ng of each expression vector according to the manufacturer’s protocol in 24-well plates. Immortalized myoblasts were transfected with 5 μg of each expression vector by electroporation using the Gene Pulser XCell (Bio-Rad) with PBS as an electroporation buffer using optimized conditions [28] . Transfection efficiencies were measured by delivering an eGFP expression plasmid (pmaxGFP, Clontech) and using flow cytometry. These efficiencies were routinely ≥95% for HEK293T and ≥70% for the immortalized myoblasts. Surveyor assay for endogenous gene modification CRISPR/Cas9-induced lesions at the endogenous target site were quantified using the Surveyor nuclease assay, which detects mutations characteristic of nuclease-mediated NHEJ. After transfection, cells were incubated for 3 or 10 days at 37 °C and genomic DNA was extracted using the DNeasy Blood and Tissue kit (QIAGEN). The target locus was amplified by 35 cycles of PCR with the AccuPrime High Fidelity PCR kit (Invitrogen) using primers specific to each locus ( Supplementary Table 5 ). The resulting PCR products were randomly melted and reannealed in a thermal cycler with the programme: 95 °C for 240 s, followed by 85 °C for 60 s, 75 °C for 60 s, 65 °C for 60 s, 55 °C for 60 s, 45 °C for 60 s, 35 °C for 60 s, and 25 °C for 60 s with a −0.3 °C s −1 rate between steps. Following reannealing, 8 μl of PCR product was mixed with 1 μl of Surveyor Nuclease S and 1 μl of Enhancer S (Transgenomic) and incubated at 42 °C for 1 h. After incubation, 6 μl of digestion product was loaded onto a 10% TBE polyacrylamide gel and run at 200 V for 30 min. The gels were stained with ethidium bromide and quantified by densitometry using the ImageLab software suite (Bio-Rad) as previously described. Fluorescence-activated cell sorting of myoblasts DMD myoblasts were electroporated with 5 μm each of hCas9-T2A-GFP and sgRNA expression vectors and incubated at 37 °C and 5% CO 2 . Three days after electroporation, cells were trypsinized and collected for FACS sorting using a FACSvantage II sorting machine. GFP-positive cells were collected and expanded for analysis. PCR-based assay to detect genomic deletions The exon 51 or exon 45–55 loci were amplified from genomic DNA by PCR (Invitrogen AccuPrime High Fidelity PCR kit) using primers flanking each locus. The flanking primers were CelI-CR1/2-F and CelI-CR5-R for exon 51 or CelI-CR6-F and CelI-CR36-R for exon 45–55 analysis ( Supplementary Table 5 ). PCR products were separated on Tris-Acetate-EDTA (TAE)-agarose gels and stained with ethidium bromide for analysis. PCR-based detection of translocations Loci with predicted possible translocations were amplified by a two-step nested PCR (Invitrogen AccuPrime High Fidelity PCR kit for each step) of genomic DNA from cells transfected with Cas9 alone (control) or Cas9 with sgRNA. In the first step, translocations that may occur at each on-target and off-target sgRNA target site were amplified by 35 cycles of PCR using combinations of Surveyor primers for each locus that were modified to include restriction sites to facilitate cloning and sequencing analysis ( Supplementary Table 5 ). One microlitre of each PCR reaction was subjected to a second round of amplification by 35 rounds of PCR using nested primer sets custom designed for each individual predicted translocation ( Supplementary Table 5 ). Each second nested PCR primer binds within the same approximate region within the primary amplicon; however, each pair was optimized using Primer3 online bioinformatics software to ensure specific detection of each translocation. PCR amplicons corresponding to the expected length of predicted translocations and only present in cells treated with sgRNA were purified (QIAGEN Gel Extraction kit) and analysed by Sanger sequencing. mRNA analysis Immortalized myoblasts were differentiated into myofibers by replacing the growth medium with DMEM supplemented with 1% insulin-transferrin-selenium (Invitrogen #51500056) and 1% penicillin/streptomycin (Invitrogen #15140) for 5 days before the cells were trypsinized and collected. Total RNA was isolated from these cells using the RNeasy Plus Mini Kit (QIAGEN) according to the manufacturer’s instructions. RNA was reverse transcribed to cDNA using the VILO cDNA synthesis kit (Life Technologies #11754) and 1.5 μg of RNA for 2 h at 42 °C according to the manufacturer’s instructions. The target loci were amplified by 35 cycles of PCR with the AccuPrime High Fidelity PCR kit (Invitrogen) using primers annealing to exons 44 and 52 to detect exon 51 deletion by CR1/5 or CR2/5 or primers annealing to exons 44 and 60 to detect exon 45–55 deletion by CR6/36 ( Supplementary Table 5 ). PCR products were run on TAE-agarose gels and stained with ethidium bromide for analysis. The resolved PCR bands were cloned and analysed by Sanger sequencing to verify the expected exon junctions. Western blot analysis To assess dystrophin protein expression, immortalized myoblasts were differentiated into myofibers as above for 6–7 days. Cells were trypsinized, collected and lysed in RIPA buffer (Sigma) supplemented with a protease inhibitor cocktail (Sigma) and the total protein amount was quantified using the bicinchoninic acid assay according to the manufacturer’s instructions (Pierce). Samples were then mixed with NuPAGE loading buffer (Invitrogen) and 5% β-mercaptoethanol and heated to 85 °C for 10 min. Twenty-five micrograms of protein were separated on 4–12% NuPAGE Bis-Tris gels (Invitrogen) with MES buffer (Invitrogen). Proteins were transferred to nitrocellulose membranes for 1–2 h in 1 × tris-glycine transfer buffer containing 10% methanol and 0.01% SDS. The blot was then blocked for 1 h with 5% milk in Tris-buffered saline with tween-20 (TBS-T) at room temperature. Blots were probed with the following primary antibodies: MANDYS8 to detect dystrophin (1:1,000, Sigma D8168) or rabbit anti-GAPDH (1:5,000, Cell Signaling 2118S). Blots were then incubated with mouse or rabbit horseradish peroxidase-conjugated secondary antibodies (Santa Cruz) and visualized using the ChemiDoc chemilumescent system (Bio-Rad) and Western-C ECL substrate (Bio-Rad). All uncropped gel images are provided in Supplementary Fig. 13 . Transplantation into immunodeficient mice All animal experiments were conducted under protocols approved by the Duke Institutional Animal Care and Use Committee. Cells were trypsinized, collected and washed in 1 × Hank’s Balanced Salt Solution (HBSS, Sigma). Two million cells were pelleted and resuspended in 5 μl 1 × HBSS (Sigma) supplemented with cardiotoxin (Sigma #C9759) immediately before injection. These cells were transplanted into the hindlimb tibialis anterior (TA) muscle of 8-week-old male NOD.SCID.gamma mice (Duke CCIF Breeding Core) by intramuscular injection. Four weeks after injection, mice were euthanized and the TA muscles were harvested. Immunofluorescence staining Harvested TA muscles were incubated in 30% glycerol overnight at 4 °C before mounting and freezing in Optimal Cutting Temperature compound. Serial 10-μm sections were obtained by cryosectioning of the embedded muscle tissue at −20 °C. Cryosections were then washed in PBS to remove the OCT compound and subsequently blocked for 30–60 min at room temperature in PBS containing 10% heat-inactivated fetal bovine serum for spectrin detection or 5% heat-inactivated fetal bovine serum for dystrophin detection. Cryosections were incubated overnight at 4 °C with the following primary antibodies that are specific to human epitopes only: anti-spectrin (1:20, Leica NCL-SPEC1) or anti-dystrophin (1:2, Leica NCL-DYS3). After primary staining, spectrin or dystrophin expression was detected using a tyramide-based immunofluorescence signal amplification detection kit (Life Technologies, TSA Kit #22, catalogue #T-20932,). Briefly, cryosections were incubated with 1:200 goat anti-mouse biotin-XX secondary (Life Technologies #B2763) in blocking buffer for 1 h at room temperature. The signal was then amplified using streptavidin-HRP conjugates (1:100, from TSA Kit) in blocking buffer for 1 h at room temperature. Finally, cryosections were incubated with tyramide-AlexaFluor488 conjugates (1:100, TSA kit) in manufacturer-provided amplification buffer for 10 min at room temperature. Stained cryosections were then mounted in ProLong AntiFade (Life Technologies #P36934) and visualized with conventional fluorescence microscopy. Deep sequencing For each of the five gRNAs, PCR was used to amplify both the target region as well as the 50 candidate off-target sites. PCR primers included Illumina TruSeq sequencing primer sequences on the 5′ ends ( Supplementary Table 6 ). A second round of PCR was then used to add Illumina flowcell binding sequences and experiment-specific indexes 5′ of the primer sequence. The resulting products were pooled and multiplex sequenced with 250 bp paired-end reads on an Illumina MiSeq instrument. Because PCR products averaged 106 bp in length, the 3′ ends of paired reads overlapped, and that overlap was used to infer complete amplicon fragments via single ungapped alignment, parameterized to score each match as 5 and each mismatch as −4. Fragments were trimmed to remove Illumina adapter and primer sequences by performing ungapped alignment (parameterized as above to allow mismatches) of paired primer sequences to fragments and retaining only sequences between primers. Trimmed fragments were aligned to the human reference genome using BLAT. Any fragment with a top-scoring alignment that was different than the expected PCR product was discarded from downstream analysis. Each of the remaining fragments was then aligned to the reference genome sequence of the expected PCR product using a global affine alignment with the following parameterization: match=5, mismatch=−4, gap open=−5, gap extend=−2. Alignments were then trimmed to the 20-bp flanking the predicted site of Cas9 nuclease activity three base pairs 5′ of the PAM; for some targets, the 20-bp window extended beyond the end of the alignment and was therefore truncated at the end of the alignment. Indel (insertion and/or deletion) statistics were gathered from these windows separately for each treatment/control following demultiplexing via sequenced barcodes, by counting gaps in the query and subject sequences of the resulting truncated alignments and tabulating numbers of fragments having any indels in these windows. Cytotoxicity assay To quantitatively assess potential sgRNA or SpCas9 nuclease-associated cytotoxicity, HEK293T cells were transfected with 10 ng of a GFP reporter and 100 ng SpCas9 expression vector and 100 ng sgRNA expression vector using Lipofectamine 2000 according to the manufacturer’s instructions (Invitrogen). The percentage of GFP-positive cells was assessed at 2 and 5 days by flow cytometry. The survival rate was calculated as the decrease in GFP-positive cells from days 2 to 5 and normalized to cells transfected with an empty nuclease expression vector as described. Accession codes: Sequencing data have been deposited in the NCBI Sequence Read Archive (SRA) under accession code SRP051210 . How to cite this article: Ousterout, D. G. et al . Multiplex CRISPR/Cas9-based genome editing for correction of dystrophin mutations that cause Duchenne muscular dystrophy. Nat. Commun. 6:6244 doi: 10.1038/ncomms7244 (2015).